High-coherence electron bunches produced by femtosecond photoionization With the development of ultrafast electron and X-ray sources it is becoming possible to study structural dynamics with atomic-level spatial and temporal resolution. Because of their short mean free path, electrons are particularly well suited for investigating surfaces and thin films, such as the challenging and important class of membrane proteins. To perform single-shot diffraction experiments on protein crystals, an ultracold electron source was proposed, based on near-threshold photoionization of laser-cooled atoms, which is capable of producing electron pulses of both high intensity and high coherence. Here we show that high coherence electron pulses can be produced by femtosecond photoionization, opening up a new regime of ultrafast structural dynamics experiments. The transverse coherence turns out to be much better than expected on the basis of the large bandwidth of the femtosecond ionization laser pulses. This surprising result can be explained by analysis of classical electron trajectories. The emerging field of ultrafast electron and X-ray diffraction creates the possibility to study physical, chemical and biological systems on a nanometre-scale with sub-picosecond time resolution. Currently, X-ray free electron lasers are able to generate intense and nearly fully coherent X-ray pulses [1] , allowing single-shot diffraction pattern recording of protein nano- and microcrystals [2] , [3] . Using femtosecond electron diffraction, atomic-level information has been obtained on the dynamics of solid-state systems [4] . Single-shot femtosecond electron diffraction experiments can be performed with photocathode sources [5] , [6] , [7] , but with a limited coherence due to the necessarily large spatial extent of the source. The coherence is sufficient to study systems of small molecules, for which ~10 4 electrons are often enough to record a diffraction pattern. However, in this way it is not possible to create electron beams with the coherence and charge (~10 6 electrons) required to measure a diffraction pattern of a protein crystal in a single shot. Proteins have large lattice constants, ranging from a few nanometre to a few tens of nanometre, are difficult to crystallize in large samples, and create complex diffraction patterns, which impose extreme beam requirements. Alternatively, high coherence DC electron beams can be created with needle-like field emission sources [8] , [9] , but these lack the required peak current. In this work an ultracold source is used, based on near-threshold photoionization of laser-cooled atoms [10] . It holds the promise to combine the best of both worlds: it is an extended source of relatively large area, allowing simultaneous extraction of the number of electrons required for recording a full diffraction pattern of a protein crystal [11] ; and it is highly coherent, owing to its low effective source temperature, which has recently been demonstrated by nanosecond photoionization [12] , [13] , [14] . The transverse coherence length of an electron beam is defined by ≡( / mc )( σ x /ε x ), with m the electron rest mass, c the speed of light, σ x the root-mean-square (r.m.s.) size of the electron beam, and ε x the transverse r.m.s. normalized emittance [15] , which is a measure for the focusability of the beam. In a beam waist, this reduces to , with the r.m.s. transverse momentum spread. To get high-quality diffraction data, should be at least a few lattice spacings a of the crystal under investigation. In principle, the coherence length can be made arbitrarily large by increasing the beam size, as ideally ε x is a conserved quantity. The proper figure of merit for coherence is therefore the relative transverse coherence length = / σ x , which can be expressed in terms of source properties: , with the r.m.s. source size and the r.m.s. transverse momentum spread at the source. The quality of the source is determined by , which for convenience is expressed in this work in terms of an effective transverse source temperature , with k B the Boltzmann constant, although typically the velocities in the electron beam do not follow a Maxwell–Boltzmann distribution. For single-shot diffraction, preferably every electron in the pulse is used, so σ x should match the size of the sample σ s , so that > a / σ s . A relative coherence length =10 −3 would, therefore, be sufficient for determining the structure of (protein) microcrystals of several thousand unit cells across. In previous experiments, the electron source temperature in the case of nanosecond near-threshold photoionization has been measured to be T =10 K, with =2 × 10 −4 ( [12] , [13] , [14] ). For femtosecond photoionization a much higher source temperature was expected, as up to now the ultracold source has always been considered as a plasma source, with a lower limit of the electron temperature determined by the spectral bandwidth of the ionization laser [11] . Assuming a Fourier-transform-limited ionization laser pulse with a full-width-at-half-maximum (FWHM) pulse duration Δ t , the electrons would then acquire a thermal distribution with . For Δ t =50 fs, this leads to a source temperature in excess of 225 K. Here we show that the actual temperature is about an order of magnitude lower, leading to electron bunches with a relative coherence length in the order of =2 × 10 −4 . This can be explained by a model that takes the dynamics of the electrons just after ionization into account, which gives rise to a transfer of kinetic energy from the transverse direction to the longitudinal direction, and thus to a much lower transverse temperature than predicted by a simple plasma model. We show that femtosecond photoionization still allows the extraction of high-coherence bunches from an extended source, opening the door to highly charged, high-coherence electron bunches and a new regime of ultrafast structural dynamics experiments. Experimental details In our experiments, electron beams are created by photoionizing laser-cooled 85 Rb atoms near the ionization threshold. Atoms are first excited to the 5 p state, and then ionized by a 58 fs FWHM long laser pulse from an optical parametric amplifier (OPA). The created electron bunches are accelerated, and pass through a magnetic lens before striking a detector. See Fig. 1 for a schematic illustration of the set-up. Additional details can be found in Methods. 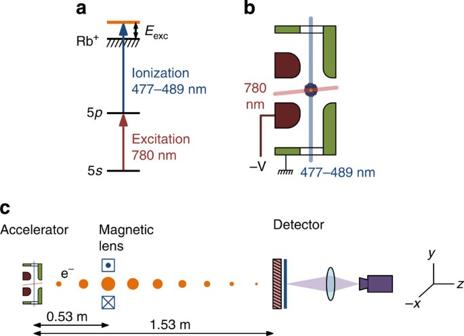Figure 1: Experimental set-up. (a) Ionization scheme. Atoms are first excited to the 5pstate, and subsequently ionized by a fs ionization laser pulse. The electrons gain an excess energyEexcin the ionization process. (b) Atoms are magneto-optically trapped inside an accelerator structure, where a part of them is ionized by two perpendicular laser beams. (c) Electron beam line. Electrons are created in the accelerator and travel to a detector, consisting of a micro-channel plate detector with a phosphor screen, which is imaged on a CCD camera. A magnetic lens is used to move the focal point of the electron beam. Figure 1: Experimental set-up. ( a ) Ionization scheme. Atoms are first excited to the 5 p state, and subsequently ionized by a fs ionization laser pulse. The electrons gain an excess energy E exc in the ionization process. ( b ) Atoms are magneto-optically trapped inside an accelerator structure, where a part of them is ionized by two perpendicular laser beams. ( c ) Electron beam line. Electrons are created in the accelerator and travel to a detector, consisting of a micro-channel plate detector with a phosphor screen, which is imaged on a CCD camera. A magnetic lens is used to move the focal point of the electron beam. Full size image For these electron beams, the normalized emittance has been determined by measuring the dependence of the beam waist at the detector on the focussing strength of a magnetic lens, a so-called waist scan. Knowledge of the source size, combined with a waist scan thus provides an upper bound for T (see Methods for details). In Fig. 2 , an example of a waist scan is shown, recorded at an ionization laser wavelength λ= 489 nm, including detector images at three particular lens currents. Those beam profiles are fitted with a rotated 2-dimensional Gaussian distribution, yielding two r.m.s. sizes per spot, which have been plotted as a function of lens current (blue squares and red circles). The two data sets have a minimum at different lens currents, as the charged particle optics suffer from astigmatism, which is accounted for in the analysis. From the fit to the data (solid curves), a source temperature T =18±4 K and a relative transverse coherence length =2.7±0.3 × 10 −4 is obtained. 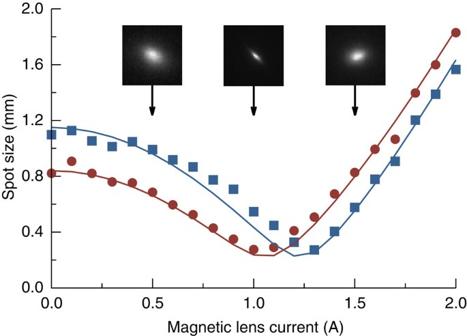Figure 2: Waist scan to determine the source temperature. The measured electron beam spot sizes (squares and circles) as a function of the current through a magnetic lens forλ=489 nm are fitted (curves) to determineT. The inset shows detector images of the electron beam for three different lens currents. Figure 2: Waist scan to determine the source temperature. The measured electron beam spot sizes (squares and circles) as a function of the current through a magnetic lens for λ =489 nm are fitted (curves) to determine T . The inset shows detector images of the electron beam for three different lens currents. Full size image Temperature measurements Using the above procedure, the source temperature has been measured as a function of the excess energy, see Fig. 3 . The excess energy E exc is the energy the electrons gain in the photoionization process (see Fig. 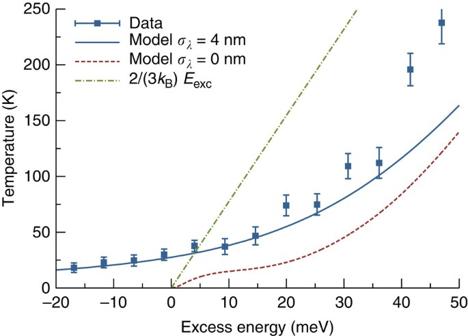Figure 3: Source temperature measurements and models as a function of excess energy. For the measurements (squares) the error bars indicate the 95% confidence bounds of the fit with equation (2). Also shown are model curves forF=0.22 MV m−1with and without taking the finite spectral width of the ionization laser into account (solid and dashed curve respectively) and the lineT=2/(3kB)Eexc(dashed-dotted curve). 1a ); it is given by the sum of the ionization energy with respect to the ionization threshold E λ in zero electric field and the Stark shift E F of the ionization threshold by the acceleration field, Figure 3: Source temperature measurements and models as a function of excess energy. For the measurements (squares) the error bars indicate the 95% confidence bounds of the fit with equation (2). Also shown are model curves for F =0.22 MV m −1 with and without taking the finite spectral width of the ionization laser into account (solid and dashed curve respectively) and the line T =2/(3 k B ) E exc (dashed-dotted curve). Full size image with λ 0 the ionization threshold wavelength (479.06 nm for 85 Rb in the 5 p state), E h =27.2 eV the Hartree energy, F the electric field strength of the acceleration field and F 0 =5.14 × 10 11 V m −1 the atomic unit of field strength. Experimentally, the excess energy is varied by changing the central OPA wavelength from 489 to 477 nm. For high excess energies, the slope of the data points equals that of the line T =2/(3 k B ) E exc , which would be implied by equipartition, but the measured temperature is significantly below this line. For low excess energies, the temperature hardly changes with excess energy. For E exc =0 meV, where half of the energy in the ionization pulse can be used to create electrons, T =30±5 K and =2.1±0.2 × 10 −4 . Analytical temperature model To explain the experimental results, a model has been developed which takes the dynamics of the electron just after the photon absorption into account, that is, its motion in the potential of the Rb + ion and the acceleration field (for a detailed description of the model, see W.E, E.V., O.L., manuscript in preparation). First the motion in a Coulomb-Stark potential is considered (sketched in Fig. 4 , solid line), for which analytic expressions exist for the classical electron trajectories in parabolic coordinates. The trajectories depend on excess energy, acceleration field strength, and starting angle β between the initial electron velocity and the direction of acceleration [16] , [17] , [18] . For E exc > E F electrons can escape the potential for any β , but for 0< E exc ≤ E F only electrons with β < β c =2 arccos(− E λ / E F ) can leave; the others represent bound states. This is illustrated in Fig. 4 , where electron trajectories are shown for different starting angles for E exc =5 meV and E F =35.8 meV, together with the corresponding potential landscape. 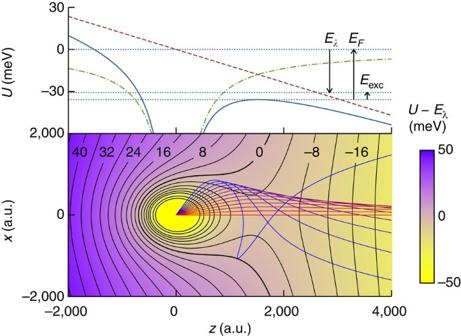Figure 4: Potential for the source temperature model. Top: Potential energyUof a combined Coulomb-Stark potential forF=0.22 MV m−1(solid curve), together with the Coulomb (dashed-dotted curve) and Stark potential (dashed curve). Bottom: Corresponding potential landscape forEexc=5 meV with equipotential lines, together with electron trajectories for different starting angles 0≤β≤βc=61°. The trajectory of the electron withβjust belowβctouches the equipotential lineU−Eλ=0 meV. a.u., atomic unit. Figure 4: Potential for the source temperature model. Top: Potential energy U of a combined Coulomb-Stark potential for F =0.22 MV m −1 (solid curve), together with the Coulomb (dashed-dotted curve) and Stark potential (dashed curve). Bottom: Corresponding potential landscape for E exc =5 meV with equipotential lines, together with electron trajectories for different starting angles 0≤ β ≤ β c =61°. The trajectory of the electron with β just below β c touches the equipotential line U − E λ =0 meV. a.u., atomic unit. Full size image This classical model of the photoionization process in an external field can be used to calculate the effective source temperature and thus the transverse coherence length. By calculating the asymptotic transverse velocity v r for electrons with a collection of starting angles, the r.m.s. transverse velocity spread can be determined. The effective temperature is then given by , which is plotted in Fig. 3 (dashed line) as function of excess energy. Because of the shape of the potential, electrons experience a force towards the z -axis when leaving the atom, thereby transferring kinetic energy in the x and y -direction to the z -direction, so and thus T <2/(3 k B ) E exc . For high excess energies, the model curve goes to the line T =2/(3 k B ) E λ , that is, the temperature is fully determined by E λ , thus independent of E F . It has been checked whether the calculated temperature changes if the Coulomb potential is replaced by a Rb model potential [19] , which takes the effect of the inner-shell electrons of Rb on the potential into account. The particle trajectories then have to be calculated by numerical simulations, using the General Particle Tracer code [20] . As the potential no longer has perfect 1/ r dependence, closed orbits no longer occur, so that electrons with β > β c can also escape the ion. This requires that at some instance such an electron approaches the ion very closely, at which point its trajectory is strongly perturbed. However, the resulting source temperatures are hardly affected. The analytic model is, therefore, used for comparison with experiments. The calculated theoretical curve T ( E exc ) (dashed curve in Fig. 3 ) has been convoluted with a Gaussian distribution corresponding to the spectral bandwidth of the femtosecond ionization laser pulse (see Methods for details). The resulting curve (solid line in Fig. 3 ) has a similar trend as the experimentally determined temperatures, but the measurement data is systematically higher. For the low excess energy regime, which is important for creating high-coherence bunches, the model curve falls within the error bars of the measurement data. The waist scan method used to determine the temperature yields an upper bound for the temperature. Any process that increases the beam size in the experiments, but is not included in the analysis, such as lens aberrations, will lead to a higher measured temperature than the actual source temperature. The work described here is an important step in realizing ultrafast electron diffraction on, for example, biologically important materials. We have shown that with 58 fs long laser pulses, electron bunches with a relative coherence length in the order of =2 × 10 −4 can be created, despite the large bandwidth of the laser pulse. This can be understood by modelling of the electron dynamics just after photoionization. The charge of the electron bunches used in this work was between 0.1 and 0.4 fC, that is, 600–2400 e − . With the peak magneto-optical trap (MOT) density being 4 × 10 16 m −3 , it would have been possible to create electron bunches with a charge of 6 fC (~4 × 10 4 e − ). This has not been done to avoid expansion of the bunch due to space charge forces. However, if the charge distribution is properly shaped [13] , space charge expansion can be reversed both transversely and longitudinally [6] . By increasing the MOT density or the size of the ionization volume in the propagation direction of the electrons, bunches can be extracted with a higher charge, without affecting the transverse coherence length. For example, with a MOT density of 10 18 m −3 ( [21] ) it is possible to extract up to 160 fC of charge (10 6 electrons) from an initial ionization volume of the same size as used in this work. One beam parameter that has yet to be measured is the pulse length, which we estimate to be dominated by two effects. Firstly, due to the finite size of the electron bunch in the accelerator, electrons are created with a longitudinal energy spread of about 0.1%, leading to a pulse length of about 25 ps at the detector. This spread also reduces the longitudinal coherence length of the bunch; however, for these electron bunches the transverse coherence is the limiting factor, and not the longitudinal coherence. Secondly, it takes the electrons a certain time to escape the Rb ion potential, which we can estimate with General Particle Tracer simulations. Electrons with starting angle β < β c will escape the potential at the first try (as in Fig. 4 ); the others will make some recursions in the potential before escaping, leading to a pulse train of electrons escaping the accelerator. The results of these simulations are comparable to experimental results [22] . When taking the bandwidth of the ionization laser into account, it is found that the electrons leave the atom in a single pulse with a pulse length of 2.5 ps FWHM for E exc =0 meV and F =0.22 MV m −1 . To get even shorter electron bunches, the resulting pulse can be temporally compressed with a radio-frequency cavity [6] , [23] , [24] . During the preparation of this manuscript, we became aware that related measurements have recently been performed using femtosecond excitation, followed by ionization with nanosecond pulses [25] . Experimental set-up Electron beams are created in three steps: First, with laser cooling techniques ~10 8 85 Rb atoms are cooled and trapped in a vapour-cell MOT resulting in a cloud with an r.m.s. radius of 1 mm. Then, the MOT is switched off for 5 μs and a part of the cloud of atoms is photoionized near the ionization threshold. Atoms are first excited to the 5 p state using a 780-nm diode laser, and then ionized by a 58 fs FWHM long, 0.46 μJ laser pulse from an OPA, pumped by a Ti:sapphire laser. The ionization laser is linearly polarized in the z -direction, the propagation direction of the electrons. We have strong indications that the polarization direction has an influence on the temperature; this is currently under investigation. Ionization only occurs where the orthogonal excitation and ionization laser beams overlap, allowing control over the initial volume size. The ionization laser wavelength λ is varied between 477 and 489 nm, with a bandwidth σ λ =4 nm. This leads to electron bunches with a charge of 0.1–0.4 fC and a transverse size of 23 × 29±2 μm. Finally, the electrons are extracted and accelerated by a DC electric field with field strength F at the acceleration point to an energy U e =0.47 eFd acc , with d acc =27 mm the effective length of the accelerator [26] , [12] . For the data presented in this work, an acceleration field of F =0.22 MV m −1 is used, leading to an electron energy U e =2.84 keV. After leaving the accelerator, the electrons pass a magnetic lens and travel a distance of 1.53 m to a micro-channel plate detector with a phosphor screen, which is imaged onto a CCD (charge-coupled device) camera. More details can be found in Ref. 12 . Source temperature determination Analogous to optical ray tracing models, a model can be constructed that describes the electron trajectories in the set-up [15] . This model relates the initial r.m.s. beam size and divergence to the final beam size ( [12] ) with M the 2 × 2 transfer matrix of the system, which can be calculated with the focal lengths and positions of the elements present in the system. The astigmatism present in the set-up is included in the transfer matrix M, giving rise to two matrices, one for each axis of the electron spot. By performing a waist scan, the effective source temperature can be determined by fitting the measured spot sizes with equation (2), with . Model temperature femtosecond pulse The analytical model provides the electron temperature as a function of the excess energy. When ionizing with a femtosecond laser pulse, electrons are created with a spread in excess energy due to the bandwidth of the laser, leading to a temperature with a normalized Gaussian weight function, the excess energy corresponding to the central wavelength of the ionization laser pulse and , where erf is the error function. How to cite this article: Engelen, W.J. et al. High-coherence electron bunches produced by femtosecond photoionization. Nat. Commun. 4:1693 doi: 10.1038/ncomms2700 (2013).